SNX13 reduction mediates heart failure through degradative sorting of apoptosis repressor with caspase recruitment domain Heart failure (HF) is associated with complicated molecular remodelling within cardiomyocytes; however, the mechanisms underlying this process remain unclear. Here we show that sorting nexin-13 (SNX13), a member of both the sorting nexin and the regulator of G protein signalling (RGS) protein families, is a potent mediator of HF. Decreased levels of SNX13 are observed in failing hearts of humans and of experimental animals. SNX13-deficient zebrafish recapitulate HF with striking cardiomyocyte apoptosis. Mechanistically, a reduction in SNX13 expression facilitates the degradative sorting of apoptosis repressor with caspase recruitment domain (ARC), which is a multifunctional inhibitor of apoptosis. Consequently, the apoptotic pathway is activated, resulting in the loss of cardiac cells and the dampening of cardiac function. The N-terminal PXA structure of SNX13 is responsible for mediating the endosomal trafficking of ARC. Thus, this study reveals that SNX13 profoundly affects cardiac performance through the SNX13-PXA-ARC-caspase signalling pathway. Heart failure (HF), the final stage of various cardiovascular diseases, is characterized by an impaired ability of the heart to fill with and/or eject blood, which is commensurate with the metabolic requirements of the body, resulting in the classic constellation of signs or symptoms of pulmonary and systemic venous congestion. HF affects ~2% of the Western population; the incidence increases from 1% in 40-year-old individuals to 10% of people above the age of 75 and is a leading cause of morbidity and mortality worldwide [1] . Despite major advances in the characterization of HF, many fundamental questions remain unanswered. Following long-standing insults, the heart undergoes protein and signal remodelling at the single-cell level in an attempt to maintain myocardial contractility and cardiac output. However, intracellular molecular remodelling may ultimately become maladaptive, leading to HF [2] . Little information is currently available regarding the molecular identity of the intracellular targeting pathways that underlie signal remodelling in failing cardiomyocytes. It is clear that transmembrane proteins, lipids and other critical cargo molecules must be selectively sorted and transported between subcellular membrane-bound compartments via membrane trafficking processes. These endocytic compartments are also critical platforms for the regulation of cell signalling, which extends well beyond the traditional function of these compartments in controlling receptor degradation [3] . Mammalian phox-homology (PX) domain-containing molecules are predominantly found in the endosomal system, where these molecules regulate diverse trafficking and signalling processes in the cell [4] . Sorting nexins (SNXs) are a particular class of PX domain-containing proteins. Different SNXs may regulate the sorting/trafficking of various proteins and may couple endosomal sorting with specific signalling events [5] . In recent years, major progress has been made in understanding the biological function and relevance of SNXs in human diseases, including cancer, pathogen invasion, inflammation and Alzheimer’s disease [6] . However, the role that SNXs play in the pathogenesis of HF remains unknown. In this study, we find that SNX13 reduction profoundly affects HF development via a mechanism that involves the lysosomal degradation of apoptosis repressor with caspase recruitment domain (ARC) and the activation of pro-apoptotic caspases. These observations suggest that SNX13 plays a crucial role in preserving cardiomyocyte survival and cardiac performance by targeting the endosomal sorting of anti-apoptotic cytoprotective signals. Endogenous SNX13 is downregulated in failing hearts To explore the potential role of SNX family molecules in HF, we performed an mRNA screen for SNX genes that might experience changes in end-stage failing human hearts. On the basis of a more profound reduction compared with all 33 SNX isoforms screened, we identified SNX13 as a candidate regulator of HF development ( Fig. 1a ). Next, we analysed the expression of SNX13 in a mouse model of HF, in which the mice underwent transverse aortic constriction or sham surgery. As shown in Fig. 1b,c , myocardial SNX13 mRNA and protein levels were clearly reduced in the mouse model of HF compared with the sham-operated control mice. These results suggested a correlation between SNX13 reduction and HF. 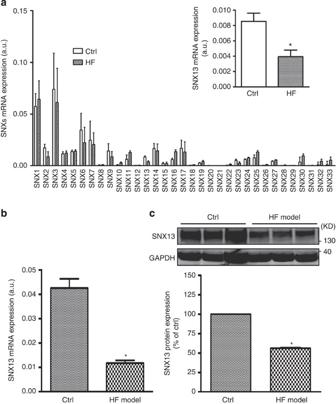Figure 1: SNX13 expression is reduced in failing hearts. (a) A quantitative PCR-based mRNA expression screen for all known SNX isoforms in end-stage failing heart tissues (N=5 per HF,N=3 per healthy control). A significant reduction inSNX13mRNA expression was identified from all 33 SNX isoforms. (b) SNX13 mRNA expression in failing cardiac tissues from experimental HF mice. (c) Western blot analysis of SNX13 protein expression in failing mice hearts (N=5 per TAC-induced HF,N=3 per sham-operated control). Ctrl, control. Data are means±s.e.m. *P<0.05 compared with Ctrl, by one-tailed unpaired Student’st-test with Welch’s correction. Figure 1: SNX13 expression is reduced in failing hearts. ( a ) A quantitative PCR-based mRNA expression screen for all known SNX isoforms in end-stage failing heart tissues ( N =5 per HF, N =3 per healthy control). A significant reduction in SNX13 mRNA expression was identified from all 33 SNX isoforms. ( b ) SNX13 mRNA expression in failing cardiac tissues from experimental HF mice. ( c ) Western blot analysis of SNX13 protein expression in failing mice hearts ( N =5 per TAC-induced HF, N =3 per sham-operated control). Ctrl, control. Data are means±s.e.m. * P <0.05 compared with Ctrl, by one-tailed unpaired Student’s t -test with Welch’s correction. Full size image Loss of SNX13 in zebrafish causes severe HF The reduction in SNX13 protein expression during HF development suggested a potential functional role for SNX13 in this process. To test this hypothesis, we examined the effect of SNX13 downregulation on cardiac function; however, SNX13 ablation is embryonically lethal in mice [7] . In contrast, zebrafish do not require a functional circulatory system during early development [8] ; thus, we used zebrafish embryos to evaluate whether in vivo SNX13 loss could cause cardiac dysfunction. The zebrafish orthologue of mammalian SNX13 was first identified by performing a BLAST search of the zebrafish Ensembl database. The zebrafish SNX13 gene encoded a protein with a high degree of identity to the human, mouse and rat SNX13 proteins ( Fig. 2a ). Next, we determined the expression of SNX13 mRNA in zebrafish embryos using whole-mount antisense RNA in situ hybridization. We found that SNX13 transcripts could be detected in the hearts of zebrafish embryos at 72 h post fertilization (h.p.f. ; Fig. 2b ). The SNX13 transcript was also expressed in heart, liver, brain and skeletal muscle tissues in adult zebrafish ( Supplementary Fig. 1 ). 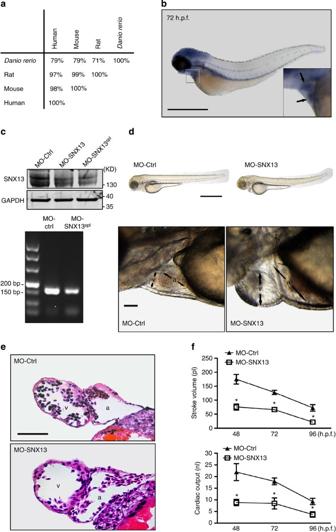Figure 2: SNX13-deficient zebrafish hearts display severe dysfunction. (a) Zebrafish SNX13 has high sequence identity with mammalian orthologues across the entire peptide sequence. (b)In situhybridization of SNX13 in the zebrafish embryos at 72 h post fertilization (h.p.f.). The rectangular box indicates the heart region. Scale bar, 500 μm. (c) Examination of SNX13 knockdown in zebrafish embryos. Upper, western blot analysis of the SNX13 protein level in MO-Ctrl-, MO-SNX13spl- and MO-SNX13-injected embryos. Glyceraldehyde 3-phosphate dehydrogenase (GAPDH) is used as the loading control. Lower, reverse transcription–PCR amplification of RNA from MO-Ctrl- and MO-SNX13spl-injected zebrafish. (d) Lateral views of zebrafish embryos at 72 h.p.f. Scale bar, 500 μm. Bottom, lateral close-up view of zebrafish hearts. The ventricular (v) and atrial (a) chambers of MO-SNX13-injected zebrafish are dilated. Scale bar, 40 μm. (e) H&E staining of zebrafish heart sections of MO-Ctrl- and MO-SNX13-injected embryos at 72 h.p.f. Scale bar, 50 μm. (f) Analysis of the stroke volume and cardiac output using high-speed laser confocal line scanning. Ctrl, control.N=32 per morphant,N=26 per MO-Ctrl. Data are means±s.e.m. *P<0.05 compared with MO-Ctrl, by one-way analysis of variance with Bonferroni’spost hoctest. Figure 2: SNX13-deficient zebrafish hearts display severe dysfunction. ( a ) Zebrafish SNX13 has high sequence identity with mammalian orthologues across the entire peptide sequence. ( b ) In situ hybridization of SNX13 in the zebrafish embryos at 72 h post fertilization (h.p.f.). The rectangular box indicates the heart region. Scale bar, 500 μm. ( c ) Examination of SNX13 knockdown in zebrafish embryos. Upper, western blot analysis of the SNX13 protein level in MO-Ctrl-, MO-SNX13 spl - and MO-SNX13-injected embryos. Glyceraldehyde 3-phosphate dehydrogenase (GAPDH) is used as the loading control. Lower, reverse transcription–PCR amplification of RNA from MO-Ctrl- and MO-SNX13 spl -injected zebrafish. ( d ) Lateral views of zebrafish embryos at 72 h.p.f. Scale bar, 500 μm. Bottom, lateral close-up view of zebrafish hearts. The ventricular (v) and atrial (a) chambers of MO-SNX13-injected zebrafish are dilated. Scale bar, 40 μm. ( e ) H&E staining of zebrafish heart sections of MO-Ctrl- and MO-SNX13-injected embryos at 72 h.p.f. Scale bar, 50 μm. ( f ) Analysis of the stroke volume and cardiac output using high-speed laser confocal line scanning. Ctrl, control. N =32 per morphant, N =26 per MO-Ctrl. Data are means±s.e.m. * P <0.05 compared with MO-Ctrl, by one-way analysis of variance with Bonferroni’s post hoc test. Full size image To inactivate SNX13 function, morpholino-modified antisense oligonucleotides directed against either the translational start site (MO-SNX13) or the splice donor sites of exon 2 (MO-SNX13 spl ) were injected into one-cell-stage zebrafish embryos. We detected an aberrant splice product in MO-SNX13 spl -injected embryos, whereas wild-type SNX13 mRNA was significantly reduced ( Fig. 2c ). A western blot analysis confirmed the effective knockdown of the SNX13 protein using MO-SNX13 or MO-SNX13 spl ( Fig. 2c ). We observed that MO-SNX13- (8 ng nl −1 ) or MO-SNX13 spl -injected (4 ng nl −1 ) embryos showed normal heart morphogenesis during the first 24 h.p.f. Between 48 and 72 h.p.f., 65% of the MO-SNX13- ( n =102) and 57% of the MO-SNX13 spl -injected ( n =95) zebrafish embryos began to develop severe HF. The injection of a mismatch morpholino (MO-Ctrl) did not lead to the MO-SNX13-specific cardiac phenotype ( n =110; data not shown). Then, we determined when HF became evident in these embryos. Compared with the MO-Ctrl siblings, these morphants demonstrated dilated atrial and ventricular chambers ( Fig. 2d ) with a decreased systolic function, as demonstrated by haematoxylin and eosin (H&E) staining of heart sections ( Fig. 2e ), by stroke volume (SV) and by cardiac output ( Fig. 2f ). The atria of MO-SNX13- and MO-SNX13 spl -injected zebrafish were also severely dilated with blood reflux from the atrium to the sinus venosus, which is another feature of congestive HF ( Supplementary Movie 1 ). Apoptosis of cardiomyocytes underlies SNX13-deficient HF To evaluate how SNX13 deficiency led to HF in the morphant embryos, we first analysed whether the disturbed structure of cardiac muscle cells was responsible. Notably, cellular autolysis, which is a form of programmed cell death, was observed in SNX13-deficient zebrafish hearts. Autolysis became more pronounced as the SNX13-deficient embryos developed beyond 72 h.p.f. ( Fig. 3a ), suggesting that cardiomyocyte death played an essential role in SNX13 deficiency-induced HF. 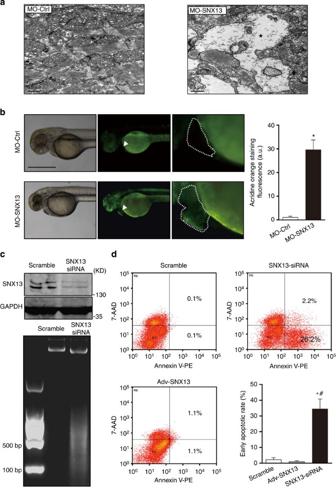Figure 3: SNX13 deficiency induces cardiac autolysis and apoptosis. (a) Transmission electron microscopy of zebrafish embryonic hearts at 72 h.p.f. Overt cardiomyocyte autolysis (black star) was observed in morphant ventricular myocytes. Scale bar, 0.5 μm. (b) AO staining of zebrafish embryos demonstrated cardiomyocyte apoptosis in SNX13 morphant hearts at 48 h.p.f. The white arrowhead and dashed line indicate the cardiac region. Right: pooled data for the AO fluorescence intensity in the cardiac area.N=6 per morphant,N=6 per MO-Ctrl. Scale bar, 400 μm. Data are means±s.e.m. *P<0.05 compared with MO-Ctrl, by one-tailed unpaired Student’st-test with Welch’s correction. (c) A DNA laddering assay in SNX13 knockdown NRVMs. Top, western blot analysis for SNX13 at 48 h after transfection with siRNA. (d) Apoptosis analysis using flow cytometry after Annexin V PE/7-AAD staining. Adv-SNX13, adenovirus-mediated SNX13 overexpression. The flow cytometry profile of a representative experiment is shown. The data were gated for damaged cells (Annexin V PE−and 7-AAD+, top left quadrant), late apoptotic cells (Annexin V PE+and 7-AAD+, top right quadrant), viable cells (Annexin V PE−and 7-AAD−, bottom left quadrant) and for early apoptotic cells (Annexin V PE+and 7-AAD−, bottom right quadrant). The percentage of early apoptotic cells was determined using flow cytometry. Ctrl, control; SNX13-wt, wild-type SNX13 overexpression.n=3. Data are means±s.e.m. *P<0.05 compared with scramble, #P<0.05 compared with groups other than scramble, by one-way analysis of variance with Bonferroni’spost hoctest.Nrepresents the number of animals, andnrepresents the number of experiments. Figure 3: SNX13 deficiency induces cardiac autolysis and apoptosis. ( a ) Transmission electron microscopy of zebrafish embryonic hearts at 72 h.p.f. Overt cardiomyocyte autolysis (black star) was observed in morphant ventricular myocytes. Scale bar, 0.5 μm. ( b ) AO staining of zebrafish embryos demonstrated cardiomyocyte apoptosis in SNX13 morphant hearts at 48 h.p.f. The white arrowhead and dashed line indicate the cardiac region. Right: pooled data for the AO fluorescence intensity in the cardiac area. N =6 per morphant, N =6 per MO-Ctrl. Scale bar, 400 μm. Data are means±s.e.m. * P <0.05 compared with MO-Ctrl, by one-tailed unpaired Student’s t -test with Welch’s correction. ( c ) A DNA laddering assay in SNX13 knockdown NRVMs. Top, western blot analysis for SNX13 at 48 h after transfection with siRNA. ( d ) Apoptosis analysis using flow cytometry after Annexin V PE/7-AAD staining. Adv-SNX13, adenovirus-mediated SNX13 overexpression. The flow cytometry profile of a representative experiment is shown. The data were gated for damaged cells (Annexin V PE − and 7-AAD + , top left quadrant), late apoptotic cells (Annexin V PE + and 7-AAD + , top right quadrant), viable cells (Annexin V PE − and 7-AAD − , bottom left quadrant) and for early apoptotic cells (Annexin V PE + and 7-AAD − , bottom right quadrant). The percentage of early apoptotic cells was determined using flow cytometry. Ctrl, control; SNX13-wt, wild-type SNX13 overexpression. n =3. Data are means±s.e.m. * P <0.05 compared with scramble, # P <0.05 compared with groups other than scramble, by one-way analysis of variance with Bonferroni’s post hoc test. N represents the number of animals, and n represents the number of experiments. Full size image Next, we used an acridine orange (AO) staining assay to indicate cells undergoing apoptosis. We compared cell death in the developing hearts of MO-SNX13-injected and scramble-injected (MO-Ctrl) embryos at 48 h.p.f. Increased numbers of AO-positive cardiomyocytes were found in MO-SNX13-injected embryos. In contrast, no cell death was detected in the atria or ventricles of scramble-injected embryos ( Fig. 3b ; Supplementary Movie 2 ). In another set of experiments, we also adopted a transgenic zebrafish line expressing the cardiac-specific myosin light chain-2 gene fused to green fluorescence protein (GFP; cmlc2:GFP) in combination with the staining of cleaved caspase-3 to show the apoptotic cardiomyocytes in the embryonic hearts. We found that the positive caspase-3 signals were observed in the cardiomyocytes of morphants but not of MO-Ctrl siblings ( Supplementary Fig. 2 ). These findings indicated that SNX13 reduction induced significant apoptosis of cardiomyocytes. Given the induction of apoptosis in SNX13-deficient zebrafish cardiomyocytes, we hypothesized that SNX13 reduction might also trigger similar events in primary mammalian cardiomyocytes. Small interfering RNA (siRNA) was used to reduce SNX13 levels in neonatal rat ventricular myocytes (NRVMs). Compared with mock control or SNX13 overexpression, the knockdown of SNX13 was sufficient to drive apoptosis, as demonstrated by DNA laddering and by fluorescence-activated cell sorting assays ( Fig. 3c,d ). These data indicated a conserved role for SNX13 in the control of cardiac cell death and survival. Extrinsic apoptosis contributes to SNX13-deficient HF To explore the effect of SNX13 deficiency-induced cardiomyocyte apoptosis on HF predisposition, we subjected wild-type and SNX13-deficient zebrafish embryos to chemical compounds known to exert antagonistic effects on critical apoptotic molecules. We determined the cardiac function after inhibiting caspase-8 (a key mediator of extrinsic apoptosis), caspase-9 (an important mediator of intrinsic apoptosis) and caspase-3 (a terminal effector for the intrinsic and extrinsic apoptotic pathways) [9] . Caspase-8 and caspase-3 inhibition markedly counteracted the cardiac cell apoptosis induced by SNX13 knockdown, whereas caspase-9 inhibition conferred a weaker effect ( Fig. 4a,b ; Supplementary Movie 3 ). Correspondingly, morphants with inhibited caspase-8 or caspase-3 underwent significant improvements in SV and in cardiac output compared with morphants with caspase-9 inhibition ( Fig. 4c ). 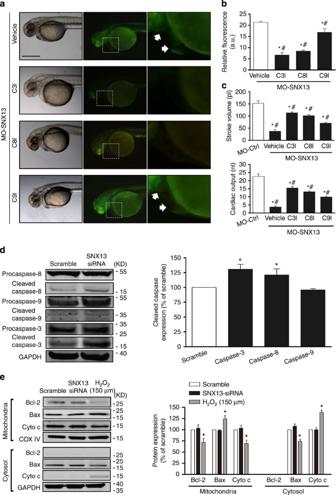Figure 4: SNX13-deficent HF links to extrinsic cardiomyocyte apoptosis. (a–c) The effects of caspase-specific inhibitory compounds (caspase-3 inhibitor Ac-DEVD-CHO, 30 μM; caspase-8 inhibitor Z-IETD-FMK, 10 μM; and caspase-9 inhibitor Z-LEHD-FMK, 20 μM) on cardiac apoptosis (a,b) and the stroke volume and cardiac output at 48 h.p.f. (c). The AO fluorescent intensity was used to evaluate apoptotic cardiomyocytes in the cardiac area (defined by arrows and outlined by dashed lines) (b).N=8 per morphant,N=10 per MO control. C3I, C8I and C9I represent inhibitors of caspase-3, -8 and -9, respectively. Scale bar, 400 μm. (d) Western blot analysis of the critical molecules of the extrinsic and intrinsic apoptotic pathways. SNX13 knockdown in NRVMs increased caspase-3 and caspase-8 expression but did not affect caspase-9 expression, as demonstrated by representative blots. Left, typical western blots; right, pooled data. (e) Western blot analysis of the protein levels of cytochromec, Bcl2 and Bax in the cytosolic and mitochondrial fractions of SNX13-deficient NRVMs. Left, typical western blots; right, pooled data. Ctrl, control.n=3. Data are means±s.e.m.*P<0.05 compared with Ctrl; #P<0.05 compared with groups other than Ctrl, by one-way analysis of variance with Bonferroni’spost hoctest.Nrepresents the number of animals, andnrepresents the number of experiments. Figure 4: SNX13-deficent HF links to extrinsic cardiomyocyte apoptosis. ( a – c ) The effects of caspase-specific inhibitory compounds (caspase-3 inhibitor Ac-DEVD-CHO, 30 μM; caspase-8 inhibitor Z-IETD-FMK, 10 μM; and caspase-9 inhibitor Z-LEHD-FMK, 20 μM) on cardiac apoptosis ( a , b ) and the stroke volume and cardiac output at 48 h.p.f. ( c ). The AO fluorescent intensity was used to evaluate apoptotic cardiomyocytes in the cardiac area (defined by arrows and outlined by dashed lines) ( b ). N =8 per morphant, N =10 per MO control. C3I, C8I and C9I represent inhibitors of caspase-3, -8 and -9, respectively. Scale bar, 400 μm. ( d ) Western blot analysis of the critical molecules of the extrinsic and intrinsic apoptotic pathways. SNX13 knockdown in NRVMs increased caspase-3 and caspase-8 expression but did not affect caspase-9 expression, as demonstrated by representative blots. Left, typical western blots; right, pooled data. ( e ) Western blot analysis of the protein levels of cytochrome c , Bcl2 and Bax in the cytosolic and mitochondrial fractions of SNX13-deficient NRVMs. Left, typical western blots; right, pooled data. Ctrl, control. n =3. Data are means±s.e.m. * P <0.05 compared with Ctrl; # P <0.05 compared with groups other than Ctrl, by one-way analysis of variance with Bonferroni’s post hoc test. N represents the number of animals, and n represents the number of experiments. Full size image We further examined whether SNX13 downregulation activated apoptotic signals in NRVMs. Western blot analysis was used to examine the expression levels of procaspases (inactivated caspases) and of cleaved caspases (activated caspases). As shown in Fig. 4d , cleaved caspase-8 and caspase-3 were elevated in NRVMs with SNX13 knockdown, whereas no significant changes in the expression of procaspase-8 and procaspase-3 were observed. We also analysed the expression of molecules that are critical to the intrinsic apoptotic pathway, including caspase-9, cytochrome c , Bcl2 and Bax. Compared with the positive control with H 2 O 2 treatment (150 μM, 6 h), SNX13 reduction did not affect the expression of pro- and cleaved caspase-9, Bcl2 or Bax ( Fig. 4e ; Supplementary Fig. 3 ). In addition, cytochrome c was not detected in cytosolic fractions of SNX13-defective NRVMs. Taken together, the SNX13 knockdown-mediated cardiomyocyte apoptosis is primarily attributed to the activation of the extrinsic apoptotic pathway. SNX13 regulates ARC-mediated cardiomyocyte apoptosis As described in the previous section, caspase-8 is a crucial signalling molecule in the extrinsic apoptotic pathway and is activated in SNX13-deficient cardiomyocytes. ARC, which is specifically expressed in striated muscles and in neurons, is a master regulator of cardiac death signalling. This molecule binds to caspase-8, inhibits its activity [10] , [11] and provides cardioprotective effects during HF development [12] . Thus, next, we investigated whether SNX13 affects caspase-8 activity by modulating the anti-apoptotic protein ARC. We performed an expression analysis of ARC in the failing hearts of experimental HF mice and in SNX13-deficient NRVMs. A significantly reduced level of the ARC protein was observed in these cells ( Fig. 5a,b ). To explore the underlying mechanism for the decreased expression of ARC in HF, ARC mRNA levels were determined using real-time PCR. The ARC mRNA levels did not differ between mouse HF hearts and related controls ( Supplementary Fig. 4a ) or between SNX13-deficient NRVMs and normal cardiomyocytes ( Supplementary Fig. 4b ), suggesting that the regulation of ARC expression occurs at the post-transcriptional level. Given the protein sorting/trafficking properties of SNX13, we investigated whether the loss of SNX13 directed ARC movement towards lysosomes and, thus, degradation. We found that the specific proteasome/lysosome inhibitor bafilomycin A1 (100 nM) [13] counteracted the ARC degradation that resulted from decreased SNX13 levels in NRVMs ( Fig. 5c ), but that proteasome inhibition with MG132 (0.5 μM) [14] did not affect ARC expression in the SNX13-deficient cardiomyocytes ( Fig. 5d ; Supplementary Fig. 5 ). In addition, RNA interference specific for LAMP1 was adopted to impair the lysosomal degradation pathway. LAMP1 depletion significantly reconciled the ARC reduction induced by SNX13 knockdown ( Fig. 5e ), which was similar to the effects of bafilomycin A1. Notably, the overexpression of ARC markedly rescued the SNX13 reduction-induced apoptosis of NRVMs ( Fig. 5f ) and the SNX13-deficient cardiac failure ( Supplementary Fig. 6 ), suggesting that SNX13 deficiency-associated apoptosis was involved in the reduced ARC levels. Taken together, these results demonstrate that SNX13 directly modulates ARC stability and that SNX13 reduction mediates the apoptotic death of cardiomyocytes by promoting ARC degradation. 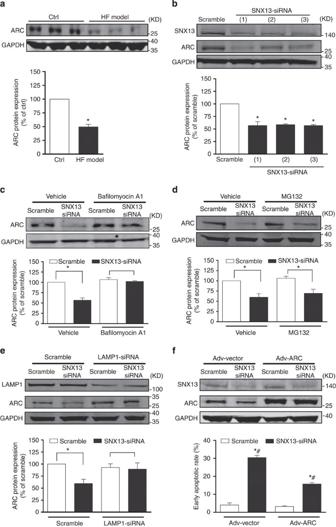Figure 5: ARC degradation mediates SNX13-deficient myocyte apoptosis. (a,b) ARC protein expression levels in failing mouse hearts and in SNX13-deficient NRVMs.n=3. Data are means±s.e.m. *P<0.05 compared with scramble, by one-way analysis of variance (ANOVA) with Bonferroni’spost hoctest. (c,d) Western blot analysis of ARC in SNX13-deficient NRVMs in the presence or absence of the lysosomal inhibitor bafilomycin A1 (Ba-A1, 100 nM) and the proteasome inhibitor MG132 (0.5 μM). Top, representative blots; bottom, quantified data. Ctrl, control.n=3. *P<0.05 compared with Ctrl or mock. (e) Effects of LAMP1 deletion on the ARC expression in SNX13-deficient cells. Top, typical western blots; bottom, quantified data. (f) Cardiomyocyte apoptosis analysis using flow cytometry after Annexin V PE/7-AAD staining. Top, western blot analysis of ARC and SNX13 proteins in NRVMs; bottom, pooled data for the apoptotic rate of NRVMs. Data are means±s.e.m. *P<0.05 compared with scramble, #P<0.05 compared with groups other than scramble, by one-way ANOVA with Bonferroni’spost hoctest. All of the data were derived from three separate experiments.nrepresents the number of experiments. Figure 5: ARC degradation mediates SNX13-deficient myocyte apoptosis. ( a , b ) ARC protein expression levels in failing mouse hearts and in SNX13-deficient NRVMs. n =3. Data are means±s.e.m. * P <0.05 compared with scramble, by one-way analysis of variance (ANOVA) with Bonferroni’s post hoc test. ( c , d ) Western blot analysis of ARC in SNX13-deficient NRVMs in the presence or absence of the lysosomal inhibitor bafilomycin A1 (Ba-A1, 100 nM) and the proteasome inhibitor MG132 (0.5 μM). Top, representative blots; bottom, quantified data. Ctrl, control. n =3. * P <0.05 compared with Ctrl or mock. ( e ) Effects of LAMP1 deletion on the ARC expression in SNX13-deficient cells. Top, typical western blots; bottom, quantified data. ( f ) Cardiomyocyte apoptosis analysis using flow cytometry after Annexin V PE/7-AAD staining. Top, western blot analysis of ARC and SNX13 proteins in NRVMs; bottom, pooled data for the apoptotic rate of NRVMs. Data are means±s.e.m. * P <0.05 compared with scramble, # P <0.05 compared with groups other than scramble, by one-way ANOVA with Bonferroni’s post hoc test. All of the data were derived from three separate experiments. n represents the number of experiments. Full size image PXA structure of SNX13 is responsible for ARC degradation To further elucidate the SNX13-dependent regulation of ARC stability in cardiomyocytes, we analysed the potential interaction of SNX13 with ARC and tracked the intracellular trafficking of ARC under SNX13 reduction in H9C2 cells, which is a permanent cell line derived from rat cardiac tissue. First, the association of SNX13 with ARC was tested using co-immunoprecipitation. Proteins in lysates from freshly isolated intact rat heart tissues were immunoprecipitated with a specific antibody against SNX13 or against ARC. SNX13 was found to co-precipitate with ARC and vice versa ( Fig. 6a ). Then, we performed immunofluorescence labelling to show the subcellular locations of SNX13 and of ARC. We observed that the endogenous SNX13 and ARC localized to early endosomes, as demonstrated by the co-localization of SNX13 and of ARC with EEA1 (a marker of early endosomes; Fig. 6b ). Identification of their expression in the purified early endosomes ( Fig. 6c ) further supported a physical interaction between SNX13 and ARC. Next, the SNX13-mediated endosomal trafficking of ARC was studied. Staining with an anti-SNX13 antibody was employed to indicate the cells with SNX13 knockdown. We found that most ARC proteins co-localized with LysoTracker (an indicator of lysosomes) in SNX13-deficient cells at 72 h after transfection with SNX13-siRNA ( Fig. 6d ). The biochemical and fluorescence microscopic data suggest that SNX13 directly interacts with ARC in the endosomes and that a reduction in SNX13 expression may facilitate the lysosomal targeting of ARC. 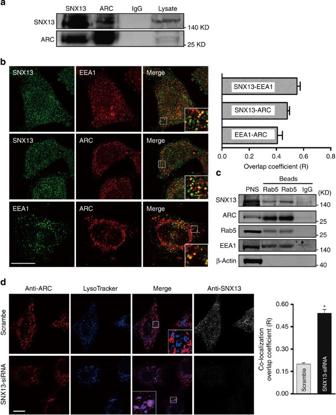Figure 6: SNX13 deficiency induces the lysosomal translocation of ARC. (a) Co-immunoprecipitation of SNX13 with ARC from NRVM lysates. (b) A representative confocal fluorescence microscopy image of the co-localization of EEA1/SNX13, EEA1/ARC and of SNX13/ARC in normal H9C2 cardiac cells. Right, pooled data showing the overlap coefficient. Scale bar, 20 μm. (c) Western blot examination of SNX13 and ARC proteins in the purified early endosomes from NRVMs. PNS, postnuclear supernatant. The representative blots were derived from three separate experiments. (d) LysoTracker and ARC images in H9C2 cells with SNX13 knockdown. Right, pooled data showing the overlap coefficient. The representative images were derived from three separate experiments. Scale bar, 25 μm. Data are means±s.e.m. *P<0.05 compared with scramble, by one-tailed unpaired Student’st-test with Welch’s correction. Figure 6: SNX13 deficiency induces the lysosomal translocation of ARC. ( a ) Co-immunoprecipitation of SNX13 with ARC from NRVM lysates. ( b ) A representative confocal fluorescence microscopy image of the co-localization of EEA1/SNX13, EEA1/ARC and of SNX13/ARC in normal H9C2 cardiac cells. Right, pooled data showing the overlap coefficient. Scale bar, 20 μm. ( c ) Western blot examination of SNX13 and ARC proteins in the purified early endosomes from NRVMs. PNS, postnuclear supernatant. The representative blots were derived from three separate experiments. ( d ) LysoTracker and ARC images in H9C2 cells with SNX13 knockdown. Right, pooled data showing the overlap coefficient. The representative images were derived from three separate experiments. Scale bar, 25 μm. Data are means±s.e.m. * P <0.05 compared with scramble, by one-tailed unpaired Student’s t -test with Welch’s correction. Full size image To gain a detailed understanding of the structural basis for the SNX13-mediated endosomal sorting of ARC, we further examined several truncated versions of SNX13 for their ability to regulate the intracellular trafficking of ARC. First, we deleted the amino-terminal PXA domain (residues 97–284), PX domain (residues 563–676), G protein signalling (RGS) domain (373–513) or carboxy-terminal PX-associated domain (PXC; 779–808; Fig. 7a ). Next, we analysed the potential interaction of ARC with these Flag-tagged mutant fusion proteins using co-immunoprecipitation. As shown in Fig. 7b , among the four truncated mutants, only the PXA-truncated mutant (ΔPXA-SNX13) could not co-immunoprecipitate with ARC, suggesting that the PXA domain may be critically responsible for the interaction between ARC and SNX13. Then, we employed a cellular imaging technique to demonstrate the subcellular localization of ARC in cells overexpressing these mutants. The mutants were transiently overexpressed in cells, and an anti-flag antibody was used to show the cells expressing these mutants ( Fig. 7c ). Immunofluorescence imaging showed that most of the tagged truncated proteins were not correctly localized to endosomes, which is different from endogenous proteins. SNX13 mutant with the N-terminal PXA domain deletion induced the lysosomal trafficking of ARC, whereas the other three truncated mutants did not affect the subcellular localization of ARC proteins ( Fig. 7c,d ), mimicking the downregulation of full-length SNX13 and suggesting that a small amount of the expressed proteins retain activity and induce the cellular phenotypes in ARC localization. Finally, we evaluated whether the overexpression of these mutants affected the activation of caspase-8, which is the direct target of ARC. Western blot examination demonstrated that ΔPXA-SNX13 overexpression increased the expression of the cleaved caspase-8 and reduced the ARC expression, as observed by SNX13 knockdown ( Fig. 7e,f ). These results indicated that the N-terminal PXA domain structure may be the decisive module for the SNX13 reduction-mediated degradative sorting of the ARC protein and for caspase activation. 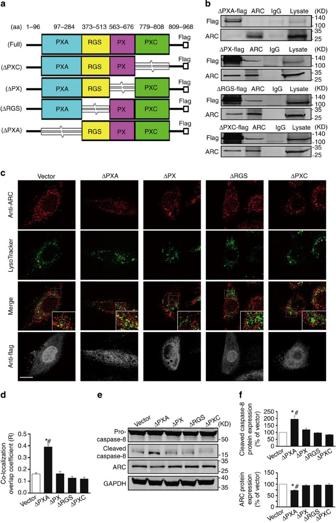Figure 7: PXA domain of SNX13 mediates intracellular ARC trafficking. (a) Scheme of the SNX13-truncated proteins. (b) Co-immunoprecipitation of ARC with different SNX13-truncated mutants. (c) Subcellular location imaging of the ARC protein at 48 h after expressing the SNX13-truncated mutants in H9C2 cells. Expression of the N-terminal PXA-truncated mutant induced the lysosomal targeting of ARC. The representative images were derived from three to five separate experiments. Scale bar, 20 μm. (d) Analysis of the co-localization of ARC with lysosomes in cells expressing different SNX13-truncated mutants. Data are means±s.e.m. *P<0.05 compared with vector control; #P<0.05 compared with groups other than vector control, by one-way analysis of variance (ANOVA) with Bonferroni’spost hoctest. (e) Typical western blot examination of the effects of SNX13-truncated mutants on caspase-8 activation and ARC expression. (f) Pooled data frome. Data are means±s.e.m. *P<0.05 compared with vector control; #P<0.05 compared with groups other than vector control, by one-way ANOVA with Bonferroni’spost hoctest. Figure 7: PXA domain of SNX13 mediates intracellular ARC trafficking. ( a ) Scheme of the SNX13-truncated proteins. ( b ) Co-immunoprecipitation of ARC with different SNX13-truncated mutants. ( c ) Subcellular location imaging of the ARC protein at 48 h after expressing the SNX13-truncated mutants in H9C2 cells. Expression of the N-terminal PXA-truncated mutant induced the lysosomal targeting of ARC. The representative images were derived from three to five separate experiments. Scale bar, 20 μm. ( d ) Analysis of the co-localization of ARC with lysosomes in cells expressing different SNX13-truncated mutants. Data are means±s.e.m. * P <0.05 compared with vector control; # P <0.05 compared with groups other than vector control, by one-way analysis of variance (ANOVA) with Bonferroni’s post hoc test. ( e ) Typical western blot examination of the effects of SNX13-truncated mutants on caspase-8 activation and ARC expression. ( f ) Pooled data from e . Data are means±s.e.m. * P <0.05 compared with vector control; # P <0.05 compared with groups other than vector control, by one-way ANOVA with Bonferroni’s post hoc test. Full size image Our study reveals that SNX13 regulates cardiomyocyte fate and cardiac performance via its N-terminal PXA domain-mediated endosomal trafficking of ARC. Five major findings that we obtained from observational clinics and from relevant experimental models support this conclusion. First, endogenous SNX13 is significantly reduced in the failing hearts of several species. Second, SNX13-deficient model organisms exhibit a striking decrease in in vivo cardiac systolic function, which is primarily linked to extrinsic apoptotic cardiomyocyte death. Third, the inhibition of cardiomyocyte apoptosis largely rescues the cardiac dysfunction associated with SNX13 reduction. Fourth, SNX13 reduction facilitates the degradation of ARC, and ARC overexpression counteracts the apoptotic death of cardiomyocytes. Fifth, the N-terminal PXA structure of SNX13 mediates the endosomal trafficking of ARC. At present, 33 mammalian SNXs have been identified. Dr Farquhar’s group was the first one to describe the SNX13/RGS-PX1 bifunctional role in the regulation of G-protein (Gαs) signalling and of endosomal sorting [15] , and successively determined that SNX13 is indispensable for embryonic development [7] . However, the role of SNX13 in the heart remains unclear. Given that the regulation of RGS proteins is reported to affect the GPCR-mediated signalling and cardiac hypertrophy [16] , SNX13 may have a potential role in the modulation of cardiac function. Our data indicate that SNX13 deficiency causes severe HF. Evidence from ultrastructural and cytochemical assays of SNX13-deficient hearts, which exhibit cellular autolysis and apoptosis, underscore the link between apoptosis and HF. Preventing apoptotic signals by inhibiting caspases largely counteracts the HF phenotype, which further establishes a prominent role for cardiomyocyte apoptosis in HF caused by SNX13 deficiency. The injury of cells or of tissues triggers cellular autolysis, which is the self-digestion or apoptosis of a cell by its own enzymes. Extensive cardiomyocyte autolysis induced by SNX13 deficiency may accelerate the loss of cardiac cells and the progression of cardiac dysfunction. Notably, the mitochondrion-dependent (intrinsic) apoptotic pathway may contribute less to the development of HF in this context; SNX13 reduction does not affect related signal markers [17] , such as cytochrome c release and Bcl2 translocation, and caspase-9 inhibition confers a weak effect against cardiac dysfunction caused by a SNX13 defect ( Fig. 4 ). Taken together, these findings indicate that SNX13 reduction-mediated HF may be caused primarily by the cardiomyocytes’ extrinsic apoptotic pathway. One of the principal mechanisms for controlling apoptosis is the regulation of protein–protein interactions [18] . As previously reported, ARC expression in the heart has cardioprotective effects against HF development. This expression blocks the intrinsic and extrinsic apoptotic death pathways by inhibiting caspase activity [12] . In the present study, our findings suggest that SNX13 physically binds to ARC and acts as an important accessory regulator of the interaction between ARC and caspase-8. Reduced SNX13 expression may disrupt ARC sorting, thereby resulting in ARC trafficking to an inappropriate cellular location for degradation, that is, the lysosome. Under these conditions, caspase-8 is activated due to the removal of ARC-mediated inhibition, leading to apoptotic cardiomyocyte death. The beneficial effects of the restoration of cardiomyocyte ARC expression on the apoptotic death caused by SNX13 reduction further confirmed the crucial role of ARC. Thus, the decreased expression of SNX13 may effectively promote cardiomyocyte apoptosis by inducing ARC degradation, leading to the development of HF. RGS proteins have been identified as important regulators of cardiovascular physiology [16] . SNX13 also serves as a guanosine triphosphatase-activating protein [15] , which may be implicated in the cardiovascular system. The intracellular cyclic AMP (cAMP) assay showed that SNX13 reduction did not affect the adrenergic receptor activation-mediated cAMP response ( Supplementary Fig. 7 ). Also, H89, which is a specific inhibitor of Gαs-mediated cAMP signalling, had no effect on aberrant cardiac function of SNX13 morphants ( Supplementary Movie 4 ). Finally, the SNX13 mutant protein lacking the RGS domain did not affect the endosomal sorting of ARC. Altogether, these results indicate that the SNX13 RGS domain is not responsible for the cardiac dysfunction associated with SNX13 reduction. In addition to the RGS domain, SNX13 possesses three other domains: N-terminal PXA, PX and PXC [5] . The PX domain is involved in the targeting of proteins to cell membranes in eukaryotes; this targeting is a hallmark feature of the SNX protein family. However, our fragment deletion approach identified that the N-terminal PXA, but not PX and the PXC structure of SNX13, mediated the endosomal sorting of ARC. Thus, the PXA module of SNX13 may be critical for the preservation of ARC recycling in the endosomal system. From a biological perspective, lysosomal turnover primarily contributes to ubiquitinated membrane protein degradation and to proteasomal turnover for cytoplasmic proteins. Several recent studies have reported that the cytoplasmic ARC protein is degraded via the ubiquitin-proteasomal pathway [19] and that an ARC ubiquitin acceptor residue mutation stabilizes and preserves its steady-state levels [20] . Our experiments with a proteasome inhibitor and with lysosome disruption suggested that the ARC protein is degraded through the lysosomal, but not proteasomal, pathway in cells with SNX13 knockdown. Thus, our present study highlights a novel mechanism for the turnover of the ARC protein. In summary, our findings suggest that a unique signalling mechanism underlies HF induced by SNX13 reduction. A novel aspect of the SNX13-dependent regulatory pathway is the determination of cardiomyocyte fate through modulating ARC turnover. SNX13 deficiency facilitates the lysosomal degradation of ARC, promoting cardiomyocyte apoptosis and HF. The manipulation of SNX13-mediated ARC stability may offer a new therapeutic strategy for HF. Human heart samples The investigation complied with the principles that govern the use of human tissues outlined in the Declaration of Helsinki. We have obtained informed consent from patients or close family members. Left ventricular samples were obtained from five explanted human hearts ( Supplementary Table 1 ). Samples were collected at the time of cardiac transplantation. Three healthy control hearts were obtained from multiorgan donors. The control hearts did not exhibit cardiovascular pathology but were unable to be used for transplantation due to technical reasons. Animal models All animal protocols were approved by the Animal Care and Use Committee at the Tongji University School of Medicine and followed the NIH Guidelines for Care and Use of Animals in Research (NIH Publication No. 85-23, revised 1996). HF models were established by transverse aortic constriction in mice. In brief, midline sternotomy was performed on mice that were anaesthetized, intubated and placed on a respirator, and 6.0 Prolene suture was placed around the aorta distal to the brachiocephalic artery. The suture was tightened around a blunt 27-gauge needle placed close to the aorta. The needle was then removed, and the chest was closed up. Echocardiography was performed at regular intervals to evaluate cardiac function using a 15-Mhz linear-array probe and a Sonos 4500 ultrasonograph (Hewlett–Packard). The animals were killed after 2 months, and the hearts were frozen in liquid nitrogen immediately on death. Zebrafish husbandry, breeding and functional assessment A wild-type AB zebrafish line was maintained at 28.5 °C in 14:10 h light/dark conditions, 50 adults per 10 l tank. To inhibit pigmentation, 0.003% 1-phenyl-2-thiourea was added to the embryo medium (17 mM NaCl, 0.21 mM KCl, 0.12 mM MgSO 4 , 0.18 mM Ca(NO 3 ) 2 , 1.5 mM HEPES, pH 7.6). The cardiac output and SV of zebrafish embryos were monitored using a high-speed confocal line-scanning microscope. Briefly, after a 3-min delay to ensure a steady-state level of anaesthesia, images were captured using a Leica SP5 laser-scanning microscope with an Olympus PlanApo N ( × 60/1.42 oil) lens using differential interference contrast (DIC) optics. Scan lines were oriented parallel to the flow of blood within the dorsal aorta, just above the yolk ball. Approximately 15,000 lines were acquired per sample at a rate of 0.488 ms per line allowing a maximum velocity of 4.10 cm s −1 to be measured. Using a 20 μm line and the optical system described above, a minimum scan rate of 8 ms per line is required to record the maximum cellular velocity of 0.25 cm s −1 observed in these experiments. Heart rates were determined by dividing 60 s by the average duration of a heartbeat, which was measured by the average peak-to-peak distance of the velocity versus time profile. SV, the volume of blood ejected by the ventricle in one heartbeat, was determined by multiplying the cross sectional area of the aorta by the distance of blood pumped along the aorta in one beat. Cardiac output, the volume of blood ejected by the heart in 1 min, was calculated by multiplying the SV by the heart rate. Morpholino microinjections A morpholino-modified oligonucleotide (Gene Tools, Philomath, OR, USA) was directed against the SNX13 translational start site (MO-SNX13: 5′-AGTTTCTCTGACATGCGGCCCATGT-3′) and the splice donor sites of exon 2 (MO-SNX13 spl : 5′-CCAGCCCCTGAATGACGGCACGGAA-3′). The morpholinos (MO-SNX13: 8 ng nl −1 ; MO-SNX13 spl : 4 ng nl −1 ) were injected into wild-type embryos at the one-cell stage. As a negative control, a standard control oligonucleotide (5′-AGTATGTCTCACATCCGCCCCATGT-3′; 8 ng nl −1 ) was injected at the same dose. Injected embryos were allowed to develop at 28.5 °C until the appropriate developmental stage. Pictures and movies were recorded at the indicated time points after the microinjection treatments. Transmission electron microscopy Embryos were fixed in 2% glutaraldehyde and 2% paraformaldehyde (PFA) in 0.1 M sodium phosphate buffer (phosphate-buffered saline (PBS); pH 7.4) overnight at 4 °C and post-fixed in 1% OsO 4 in PBS (pH 7.2). Fixation was followed by staining with 5% uranyl acetate in H 2 O for 1 h and then dehydrated by serial steps in ethanol, embedded in Epon and polymerized at 60 °C for 24 h. Ultrathin sections (70–90 nm) were cut, then stained with uranyl acetate or alternatively stained with lead citrate and uranyl acetate. The sections were analysed under a JEM-1230 transmission electron microscope. Recombinant adenovirus construction and transfection For recombinant adenovirus construction, the rat SNX13 complementary DNA (cDNA; Ad-SNX13) and the GFP gene (Ad-GFP; control) cloned by PCR was inserted into pDC315-EGFP vector (purchased from Hanbio, Shanghai, China) under the control of the rat cytomegalovirus promoter. The pDC315-SNX13 and pBHGloxE1,3 Cre were co-transfected into HEK293 cells by using LipoFiter transfection reagent (Hanbio) to generate the recombinant adenoviruses. Ad-SNX13 and Ad-GFP were propagated in HEK293 cells. The propagated recombinant adenoviruses in the HEK293 cells were purified and the titre of virus was measured by plaque assays. The stock solutions of Ad-SNX13 and Ad-GFP were 1 × 10 10 plaque formation unit ml −1 . Cardiomyocytes were kept in serum-free medium (control medium) supplemented with transferrin (5 mg ml −1 ) and insulin (1 mg ml −1 ) for 24 h before adenoviral infection. NRVM isolation and transfection Single cardiac myocytes from the hearts of 2–3-day-old Sprague Dawley rats were isolated by digestion with collagenase. Briefly, ventricles from neonatal rats were cut into pieces and then dissociated in calcium-free HBSS containing 0.125 mg ml −1 trypsin (Gibco) and 10 μg ml −1 DNase II (Sigma). Digestion was performed at 37 °C in eight to ten 5-min steps, collecting the supernatant to fetal bovine serum (FBS; Gibco) after each step. The collected supernatant was centrifuged and resuspended in DMEM (Gibco) supplemented with 10% FBS and with 100 μM BrdU (5-bromodeoxyuridine; Sigma). The collected cells were passed through a cell strainer (100 mm, BD Falcon) and then seeded onto 100-mm plastic dishes for 2 h at 37 °C in 5% CO 2 and humidified atmosphere. The supernatant was then collected and plated onto 1% gelatin (Sigma)-coated dishes. The next day, the medium was changed by DMEM (Gibco) with 2% FBS (Gibco), 1% insulin-transferrin-selenium (ITS) (Gibco) and 100 μM BrdU (Sigma). SNX13-siRNA and LAMP1-siRNA were transfected by using Lipofectamine RNAiMAX (Invitrogen). siRNA sequences for SNX13 are as follows: (1) 5′-CAGCCGGUGAUGAUUAUAUTT-3′ and 5′-AUAUAAUCAUCACCGGCUGTT-3′; (2) 5′-GAGGCCUUUAUGAACAUUATT-3′ and 5′-UAAUGUUCAUAAAGGCCUCTT-3′; and (3) 5′-CCGAGCUUGACAUGUUAAATT-3′ and 5′-UUUAACAUGUCAAGCUCGGTT-3′. siRNA sequences specific for LAMP1 is as follows: 5′-GGGUCUACAUGAAGAAUGUTT-3′ and 5′-ACAUUCUUCAUGUAGACCCTT-3′. MG132 (0.5 μM, Sigma) or bafilomycin A1 (100 nM, Sigma) was added to culture medium for 48 h just following SNX13-siRNA transfection. Mitochondrial protein extraction For mitochondrial protein analysis, the mitochondria of cardiomyocytes were isolated using mitochondria isolation kit (Sigma). Cross-contamination of cytosol and mitochondria was determined on the basis of the amount of activity of marker enzymes for cytosol (GAPDH) and mitochondria (succinate dehydrogenase). Protein levels in the samples were determined with Bio-Rad protein assay kit. Immunocytochemistry and immunofluorescence microscopy Cells were grown at low density on coverslips for indicated time before being processed for immunocytochemistry. They were fixed in 4% PFA for 15 min at room temperature, permeabilized in PBS containing 0.01% Triton X-100 (Sigma) for 10 min and incubated with 1% bovine serum albumin (BSA) in PBS with Tween 20 (PBST) for 30 min to block unspecific binding of the antibodies. The permeabilized cells were then incubated with primary antibodies (ARC: 1/100, ab126238, Abcam; SNX13:1/100, ab67361, Abcam; EEA1:1/300, ab2900, Abcam; Flag: 1/500, F1804, Sigma) for 1 h at room temperature or overnight at 4 °C in PBST containing 1% BSA, and washed three times in PBS. After the cells were incubated for 1 h at room temperature with secondary antibodies (1/300, Invitrogen) and washed three times in PBS, cells were analysed with a Leica SP5 confocal microscope using a × 63 fluorescence lense. For lysosome labelling, cells were first incubated with 150 nM Lysotracker (Invitrogen) in culture medium for 30 min at 37 °C. Co-localization was analysed by using ImagePro Plus software. Histologic sections, H&E staining and in situ hybridization Embryos were fixed with 4% PFA overnight at 4 °C and mounted in 1% agarose. The agarose block was gradually dehydrated with 70, 90, 100% ethanol and 100% xylene and embedded in paraffin. The embryos were cut into 7 μm sections, which were stained with H&E. For whole-mount in situ hybridizations, digoxigenin-labelled riboprobes for SNX13 were synthesized from cDNA as run-off transcripts from linearized templates by using the Genius System DIG RNA Labeling Kit. Probes were detected using an alkaline phosphatase-conjugated antibody and visualized with 4-nitroblue tetrazolium/5-bromo-4-chloro-3-indolyl phosphate (NBT/BCIP; Roche Molecular Biochemicals, Indianapolis, IN, USA). Embryos were analysed using a LeicaM205FA microscope. Detection of cell death To detect apoptotic cells in live embryos, embryos were dechorionated and soaked in egg water containing 2 μg ml −1 AO at 28 °C for 30 min. After washing with egg water for eight times, embryos were anaesthetized with tricaine, mounted in 2% methylcellulose and examined by stereomicroscopy. To determine whether apoptosis was localized to cardiomyocytes, a transgenic zebrafish line expressing the cardiac-specific light myosin 2 (cmlc2) was employed. The transgenic embryos were further used for the analysis of apoptosis by whole-mount immunofluorescence to detect activated caspase-3. Briefly, zebrafish embryos were collected in a Petri dish in 1 × egg water. Then, up to 40 embryos were transferred to a 1.5-ml tube and rinsed two times with 1 ml of 1 × PBST. After removing PBST, 1 ml of 4% PFA was added and the tubes were placed on a gentle rocker at 4 °C overnight. Following the fixation, embryos were treated with 100% ice-cold methanol (1 ml) at −20 °C for 2 h and subsequently washed with fresh PDT (1 × PBST, 1% DMSO, 0.3% Triton-X) for 30 min. Finally, 1 μl rabbit anti-activated caspase-3 antibody (1:100, C8487, Sigma) was added with the appropriate dilution of an anti-rabbit fluorophore-conjugated antibody that absorbs blue light and emits green light. After addition of the secondary antibody, embryos were kept in dark for analysis. Reverse transcription–PCR Heart, liver, muscle and brain tissues were separated from adult zebrafish, and mRNA was extracted from the pooled tissue using TRIzol reagent (Invitrogen). For the subsequent PCR, the following protocol was used: 4 μl buffer, 2 μl MgCl 2 , 1 μl deoxy-ribonucleoside triphosphate (dNTP) (10 mmol l −1 ), 1 μl of each primer (20 μmol l −1 ), 8 μl cDNA, 0.5 μl (2.5 U) AmpliTaq Gold polymerase and 32.5 μl H 2 O. PCR was performed at 94 °C for 2.45 min, followed by 63 cycles at 94 °C for 0.45 min, 57 °C for 0.45 min and 72 °C for 0.45 min. The reverse transcription–PCR primer sequences were as follows: DaSNX13-RT-F (5′-GTTGAAGCACATCATCGGCG-3′) and DaSNX13-RT-R (5′-GGAACAGCGTCTCCAGGAAG-3′). After a final extension of 72 °C for 7 min, the PCR products were electrophoresed on a 1.8% agarose gel and ethidium bromide stained. Western blot analysis Ventricular tissue or myocytes were lysed in radioimmunoprecipitation buffer (50 mM Tris, 150 mM NaCl, 1 mM Na 2 -EDTA, 1% Triton X-100, 1% sodium deoxycholate, 2 mM NaF and 200 μM Na 3 VO 4 at pH 7.4). The lysates were heated to 95 °C, size fractionated in NuPAGE gels (Invitrogen) and transferred to polyvinylidene fluoride membranes. The membranes were blocked with 5% skim milk for 1 h and incubated overnight at 4 °C with the appropriate primary antibodies: SNX13 (1:1,000, AP12244b, Abgent), ARC (1:1,000, NBP1-76952, Imgenex), GAPDH (1:1,000, AG019, Beyotime), caspase 8 (1:1,000, AC056, Beyotime), caspase 9 (1:1,000, AC062, Beyotime), caspase 3 (1:1,000, AC031, Beyotime), Bcl-2 (1:1,000, AB112, Beyotime), Bax (1:1,000, 5,023, Cell Signaling), cytochrome c (1:1,000, 11,940, Cell Signaling), COXIV (1:1,000, AC610, Beyotime), LAMP1 (1:1,000, ab13525, Abcam), Rab5 (1:1,000, Cell Signaling), EEA1 (1:1,000, ab2900, Sigma), β-actin (1:1,000, AA128, Beyotime) and flag (1:1,000, F1804, Sigma). After incubation with horseradish peroxidase-conjugated secondary antibodies for 1 h at room temperature, the immunoblots were visualized using enhanced chemiluminescence (Pierce). Band intensities were analysed using Quantity One image software (Bio-Rad). Uncropped scanned images of western blots are presented in Supplementary Fig. 8 . Flow cytometry After transfecting for 48 h, the myocytes were stained with Annexin V PE and 7-aminoactinomycin D (7-AAD) (Annexin V PE Apoptosis Detection Kit PE, eBioscience) and analysed using flow cytometry (Beckman Coulter). The data were expressed as percentages of the total cell population. Immunoisolation of Rab5-positive endosomes NRVMs were washed with PBS at 4 °C and suspended in homogenization buffer (3 mM imidazole, 250 mM sucrose, 0.5 mM EDTA and complete EDTA-free protease inhibitor cocktail; Roche Diagnostics, IN). Cells were homogenized and centrifuged for 10 min at 3,000 r.p.m. The resulting postnuclear supernatant was adjusted to 40.6% sucrose, placed in 14-ml capacity ultra-clear centrifuge tubes (Beckman), overlaid with 6 ml of 35% sucrose and 4 ml of 25% sucrose and then centrifuged in a SW 41Ti rotor at 108,000 g for 3 h at 4 °C. The endosome-enriched fraction at the 25–35% sucrose interface was collected. Rabbit anti-Rab5 (1:50, 3,547, Cell Signaling) or a nonspecific rabbit IgG (Immunoglobulin G; 1:50, I5006, Sigma) was added and incubated with the isolated endosomes overnight at 4 °C with rotation. In addition, 50 μl Dynabeads (Invitrogen) were washed three times and incubated with 1 ml PBS containing 1% BSA overnight at 4 °C. The following day, the beads were recovered, added and incubated with Rab5 antibody or IgG-endosome fractions for 6 h at 4 °C with rotation. The bead–antibody–endosome complexes were collected and washed twice. Then, the samples were analysed by 10% SDS–PAGE and immunoblotting. Immunoprecipitation analysis Adult rat ventricles were cut into small pieces and homogenated in lysis buffer. After centrifugation, the supernatants were collected and incubated overnight at 4 °C with primary antibodies SNX13 (1:50, AP12244b, Abgent) and ARC (1:50, NBP 1-76952, Imgenex) by constant stirring. In addition, 50 μl Dynabeads (Invitrogen) were incubated with 1 ml 1% BSA/PBS overnight at 4 °C. The following day, the beads were recovered, added and incubated with the antibodies for 6 h at 4 °C with rotation. The bead–antibody complexes were collected and washed twice. Then, the samples were analysed by 10% SDS–PAGE and immunoblotting. DNA ladder analysis To detect DNA fragmentation, genomic DNA was isolated from NRVMs using a DNA Isolation Kit (Puregene) and resolved on a 1.5% agarose gel. DNA construction For expression of recombinant proteins in mammalian cells, different truncated fragments of human SNX13 were subcloned into the expression vector Flag (Clontech, Palo Alto, CA, USA). cDNAs encoding SNX13 fragments were derived by PCR. These constructs were transformed into Escherichia coli DH5α cells (Tiangen, Shanghai, China) and were screened by PCR with the corresponding primers for each construct. Positive colonies were selected, and the correct inserts were confirmed by DNA sequencing. DNA constructions were transfected into isolated myocytes by using Lipofectamine 2000 (Invitrogen) and analysed by 10% SDS–PAGE and immunoblotting. Cell lysates were collected for immunoprecipitation analysis by using primary antibodies flag (1:50, F1804, Sigma) and ARC (1:50, NBP 1-76952, Imgenex). Fluorescence resonance energy transfer measurement Neonatal rat cardiomyocytes transfected by PKA biosensor ICUE1 (provided by Dr Jin Zhang, Johns Hopkins University School of Medicine) were rinsed and maintained in PBS with calcium for fluorescence resonance energy transfer recording. Cells were imaged on a Zeiss Axiovert 200 M microscope with a cooled charge-coupled device camera. Dual-emission ratio imaging was acquired with a 420DF20 excitation filter, a 450DRLP dichroic mirror and two emission filters (475DF40 for cyan and 535DF25 for yellow). Exposure time was 200 ms, and images were taken every 8 s. Images in both channels were subjected to background subtraction, and ratios of cyan-to-yellow colour were calculated at different time points. cAMP assay Cardiomyocytes’ intercellular cAMP concentration was detected by using cAMP-Glo Assay kit (Promega). Briefly, after transfection with SNX13-siRNA or scramble for 48 h, cardiomyocytes were trypsinized, washed and distributed equally to a 96-well assay plate with white clear bottom. On day 2, medium was changed with 1 μM isoproterenol induction buffer for 30 min, and then the cell intercellular cAMP concentration was measured according to the assay kit protocol. The cAMP accumulation after isoproterenol treatment of the SNX13-siRNA group was compared with the control group. Measurement of proteasomal activity Proteasome activity was analysed by Proteasome-Glo Chymotrypsin-Like Cell-based Assay Kit (Promega). Briefly, NRVMs were treated with 0.5 or 1 mM MG132 for 48 h, and then cells were trypsinized, washed twice by PBS and counted to optimize cell number for a 96-well plate. The proteasome activity was measured following the assay kit protocol. Statistical analysis All data are expressed as the mean±s.e.m. In all experiments, N represents the number of animals, and n represents the number of experiments. An unpaired t -test with Welch’s correction or a one-way analysis of variance is used to compare experimental groups with their appropriate control unless otherwise specified; P <0.05 is considered significant for all experiments. How to cite this article: Li, J. et al. SNX13 reduction mediates heart failure through degradative sorting of apoptosis repressor with caspase recruitment domain. Nat. Commun. 5:5177 doi: 10.1038/ncomms6177 (2014).